A reversible conversion between a skyrmion and a domain-wall pair in a junction geometry Skyrmions are expected to be a key component of the next-generation of spintronics: known as ‘skyrmionics’. On the other hand, there is a well-established memory device encoded by a sequence of domain walls. Here we show a conversion is possible between a skyrmion and a domain-wall pair by connecting wide and narrow nanowires, enabling the information transmission between a skyrmion device and a domain-wall device. Our results will be the basis of a hybrid device made of skyrmions and domain walls, where the encoded information in domain walls is converted into skyrmions, and then read out by converting the skyrmions back to domain walls after a functional control of the skyrmions. Such a device has the potential to outperform domain-wall racetrack memory because of the combined advantages of domain walls and skyrmions for spintronics application. Skyrmion is a topological object in continuum field theory [1] . It was originally introduced in the context of nuclear physics to describe a certain particle-like configuration. The concept has now been used widely in condensed matter physics including quantum Hall ferromagnets, Bose–Einstein condensates, crystalline liquids and chiral magnetic materials [2] , [3] . Recent experimental observation of skyrmions in chiral ferromagnet evokes a flourish of its extensive study [3] , [4] , [5] , [6] , [7] , [8] , [9] , [10] , [11] , [12] , [13] , [14] , [15] . It is stabilized dynamically by the Dzyaloshinskii–Moriya interaction (DMI) and external magnetic field [16] , [17] , [18] , [19] , [20] . Once it is created, its stability is topologically protected against dissipation and fluctuation even in the presence of large defects [2] , [21] . A skyrmion can be moved along the transmission channel (for example, a nanowire) by applied electric current through the spin transfer torque (STT) mechanism. Indeed, a train of skyrmions in magnetic perpendicular magnetic anisotropy (PMA) nanotrack with DMI has been proposed to be a novel alternative as an information carrier [2] , [21] , which is called ‘skyrmionics’. However, the generation of an isolated skyrmion remains a challenging task [21] , [22] , as it is impossible to change continuously the topological number from zero to its quantized value. This is only true in the limit of continuum description. For real magnetic systems, the topological objects may simply be driven out of the edge of the nanostructures. In addition, once the continuity of the field is broken by such as applying a laser beam [23] , [24] or applying a circulating current [25] , we can create a skyrmion. A skyrmion can also be created or destroyed when it touches an edge of the sample as the spins can rotate at the edge. A recent theoretical study has shown that a skyrmion can be created from the notch of a nanowire by applying an electrical current [22] . Nonetheless, the stability of skyrmion in finite system (including nanowire or nanodisk) is still much more enhanced as compared with non-topological objects, thanks to its topological protection. On the other hand, current-induced domain wall (DW) motions in magnetic thin film have been extensively studied in recent years for potential applications in high-efficiency and low-dissipation spintronic memory. Many novel concepts and designs based on current-driven DW motions have been proposed theoretically and realized experimentally including the racetrack memory, where a train of DWs are moved along a nanowire, for ultradense information storage and information processing [26] , [27] . DW in ultrathin magnetic films layered between a heavy metal and an oxide with PMA [28] , [29] , [30] , [31] shows anomalously large velocity under current-induced STT. Such intriguing results generated competing explanations of their underlying physical mechanisms [28] , [29] , [32] , [33] . More recently, chiral DWs with a preferred handedness that is influenced by DMI have been observed, which have sparked wide interest for emerging spintronics applications based on chiral magnetism [34] , [35] , [36] , [37] . Although DW spintronics has attracted much interest for the potential applications of ultrahigh-density information-processing devices, the central issues are further reduction of the power consumption and the joule heating. It is important that both skyrmions and DWs are accommodated albeit different geometries in non-centrosymmetric bulk materials or thin film heterostructure lacking inversion symmetry. Here, we focus on the following issues of a DW pair and a skyrmion: (a) Is it possible to realize the integration of DW and skyrmion devices, such that they can be mutually converted to each other in one system? (b) Is it possible to combine important properties and advantages of these two very different magnetization textures? Our answers are affirmative. We present an explicit conversion mechanism between a skyrmion and a DW pair by employing nanowires with different widths. We propose a hybrid functional device where the information is encoded as a train of DWs and then converted into a train of skyrmions. After a functional control of the skyrmions, the information is read out by converting the skyrmions back to the DWs. It is intriguing that we can also generate a half-skyrmion (meron) from a DW pair. It has one half of the skyrmion number. Such a topological object is known as a vortex in magnetic system with disk geometry [38] . The reason why a fractional topological number is allowed reads as follows: a half-skyrmion is attached to a wall in our case, whereas a vortex [38] is confined within a disk geometry where the spin is out-of-plane at the centre but in-plane at the disk boundary because of the dipole–dipole interaction (DDI). In this way, a rich variety of topological objects are possible in magnetic system by controlling the geometry. Model and simulations The micromagnetic energy density of the system in the continuum approximation is given by where m ( r ) represents the local magnetic moment orientation (that is, | m ( r )|=1), and μ denotes its cartesian component. A ex represents the ferromagnetic exchange strength. H app is the applied magnetic field. K u is the effective uniaxial anisotropy constant with e z representing the easy-axis (that is, PMA). μ 0 is the vacuum permeability. M s represents the saturation magnetization. H dd is the magnetic DDI shown in the Methods. There exist two types of DMI, depending on samples [2] , [16] , [17] . The last term in equation (1) with strength D represents the Neel-type DMI, whereas the Bloch-type DMI has the form of m ( r )·[ ∇ × m ( r )]. It determines how spins cant at the edge of a sample and how spins swirl around the skyrmion core. In this work, we assume the Neel-type (hedgehog) skyrmion, and we have checked the results remain essentially the same for the Bloch-type (vortex-like) skyrmion. We have numerically solved the Landau–Lifshitz–Gilbert equation, which governs the dynamics of the magnetization m i at the lattice site i , where γ is the gyromagnetic ratio and α is the Gilbert-damping coefficient originating from spin relaxation. The coefficient β of the fourth term determines the strength of the non-adiabatic torque. a is the lattice constant and p is the spin polarization of the electric current. The effective magnetic field acting on the local magnetization m i includes the contribution from the Heisenberg exchange, DMI, PMA, DDI field and the applied magnetic field. The third term describes the coupling between the spin and the spin-polarized electric current j ( r ) via STT, whereas the fourth term via non-adiabatic effects. The current density in the wide and narrow parts of the wire is inversely proportional to their individual width, that is, w n / w t , where w n and w t represent the width of the narrow and wide parts of the nanowire, respectively. We have additionally included DDI in all numerical calculations [39] . However, the results remain quantitatively the same as those without the DDI. All micromagnetic simulations are performed without applying magnetic field unless otherwise specified. For finite temperature simulation shown in the Supplementary Fig. 13 , we include the stochastic thermal field term (Gaussian white noise) in the effective field (see Methods). Open boundary conditions are used for the sample edges. The nanowire is assumed to be a 1-nm thick Cobalt on a substrate inducing DMI. The length of the nanowire is 800 nm. Although the width of the right half of the nanowire ( x ⩾ 400 nm) is fixed to be 100 nm, the left part ( x <400 nm) is varied between 10 and 80 nm. The following material parameters are adopted [21] : A ex =15 pJ m −1 , α =0.3, M s =580 kA m −1 , D =3 mJ m −2 and K u =0.7 mJ m −3 . In Supplementary Notes 1–5 and Supplementary Figs 1–13 , we have also demonstrated the main conclusion of this work holds for a wide range of material parameters. All of our simulations are performed with unit cell size of 1 nm, which is sufficiently smaller than the typical exchange length scale and the skyrmion size to ensure the numerical accuracy. For simplicity, the non-adiabatic torque coefficient β is set to the same value as the Gilbert-damping constant α so that a skyrmion moves along the central line of the nanotrack without additional transverse motion [21] . Actually, the skyrmion can still travel along the nanowire even when β is not exactly equal to α , thanks to the skyrmion-edge repulsive effect [21] , [22] , [40] . Moreover, even when α ≠ β , similar results are obtained provided β is not too different from α (see Supplementary Note 5 and Supplementary Fig. 12 ). Skyrmion and topological stability A magnetic skyrmion is a texture of the normalized classical spin m =( m x , m y , m z ), which has a quantized topological number. The ground-state spin at the outer periphery is up, that is, (0, 0, 1), whereas the spin direction of the skyrmion centre is down, that is, (0, 0, −1). Spins swirl continuously around the core and approach the ground-state value asymptotically. The skyrmion is characterized by the Pontryagin number Q , which is the topological number in the planar system, Q =∫ dxdyρ sky ( x ), with We obtain Q =1 for a skyrmion in a sufficiently large area. Consequently, even if the skyrmion spin texture is deformed, its topological number does not change. It can be neither destroyed nor separated into pieces, that is, a skyrmion is topologically protected. The necessary conditions of the topological conservation are the continuity of the spin texture and the boundary condition imposed on it. On one hand, the continuity of the spin texture is destroyed for instance by applying a laser or considering a microscopic phenomenon comparable with the lattice constant. On the other hand, when a skyrmion touches an edge of the sample, the topological number may continuously change. Then we can create or destroy a skyrmion. The main topic of this work is the demonstration of mutual conversion between a skyrmion, which is a topological object ( Q =1), and a DW pair, which is non-topological object ( Q =0). Once the skyrmion is created and moves into a sufficiently large sample without touching the edge, it is a stable object due to its topological protection. Creation of skyrmion from DW and vice versa Chiral DWs are expected for a magnetic PMA thin film on a substrate inducing DMI. Chiral structures such as skyrmions are also stabilized in such a system. We consider a nanowire geometry with the width W . A skyrmion has an intrinsic radius R =28 nm determined by the material parameters and nanowire geometry. A skyrmion is stable for W >2 R , whereas it cannot exist for W <2 R , and the resultant structure will be a DW pair. We investigate a junction comprised of a narrow nanowire ( W <2 R ) on the left side and a wide nanowire ( W >2 R ) on the right side: see Fig. 1a . By applying a spin-polarized current from the right to the left, a DW pair moves in the opposite direction and then is converted into a skyrmion ( Supplementary Movie 1 ). 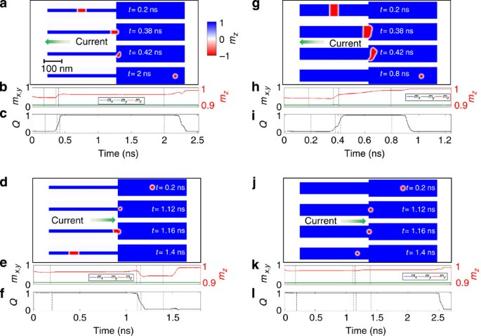Figure 1: Conversion between a skyrmion and a DW pair. (a–c) A DW pair is converted into a skyrmion driven by STT from the narrow part to the wide part of the nanowire. (a) The snapshots of the magnetization configuration at four selected times corresponding to the four vertical lines inbandc. The in-plane current density along −xdirection is 1.8 μA nm−2in the wide part. (b) The time evolution of the average spin componentsmx,my,mz. (c) The time evolution of the Pontryagin numberQ. (d–f) Reverse process ofa–c. The in-plane current density along +xdirection is 1.8 μA nm−2in the wide part. (g–i) Conversion process of a DW pair into a skyrmion similar toa–c, when the width of the narrow part is larger than the skyrmion intrinsic size. The in-plane current density along −xdirection is taken as 6.6 μA nm−2in the wide part so that the current density in the narrow part ing–iis the same as that ofa–c. (j–l) Reverse process ofg–i, where a skyrmion is not converted into a DW pair. The in-plane current density along +xdirection is 1.8 μA nm−2in the wide part. For all simulations, the initial magnetization is assumed to align along +zexcept that the magnetization inside the DW pair (or skyrmion core) are aligned −z. During the first 0.2 ns, the system is relaxed to an energy minimum state without applying any current. The colour-scale shown betweenaandghas been used throughout this paper. A physical length scale bar is included ina. Figure 1: Conversion between a skyrmion and a DW pair. ( a – c ) A DW pair is converted into a skyrmion driven by STT from the narrow part to the wide part of the nanowire. ( a ) The snapshots of the magnetization configuration at four selected times corresponding to the four vertical lines in b and c . The in-plane current density along − x direction is 1.8 μA nm −2 in the wide part. ( b ) The time evolution of the average spin components m x , m y , m z . ( c ) The time evolution of the Pontryagin number Q . ( d – f ) Reverse process of a – c . The in-plane current density along + x direction is 1.8 μA nm −2 in the wide part. ( g – i ) Conversion process of a DW pair into a skyrmion similar to a – c , when the width of the narrow part is larger than the skyrmion intrinsic size. The in-plane current density along − x direction is taken as 6.6 μA nm −2 in the wide part so that the current density in the narrow part in g – i is the same as that of a – c . ( j – l ) Reverse process of g – i , where a skyrmion is not converted into a DW pair. The in-plane current density along + x direction is 1.8 μA nm −2 in the wide part. For all simulations, the initial magnetization is assumed to align along + z except that the magnetization inside the DW pair (or skyrmion core) are aligned − z . During the first 0.2 ns, the system is relaxed to an energy minimum state without applying any current. The colour-scale shown between a and g has been used throughout this paper. A physical length scale bar is included in a . Full size image Figure 1b shows the time-evolution of the average magnetization m =( m x , m y , m z ). m x and m y are almost zero between 0< t <0.2 ns during the relaxation process. At t =0.2 ns, the finite (but still very small) in-plane spin emerges because of the STT from the injected current. Figure 1c shows the Pontryagin number changes continuously between one for a skyrmion and zero for a DW pair. The Pontryagin number can change its value when it interferes with an edge. The main message is that a skyrmion and a DW pair can be transformed continuously. A skyrmion is destroyed when it touches the sample edge. Accordingly, the Pontryagin number becomes zero after the skyrmion is expelled from the right edge of the sample ( Supplementary Movie 1 ). Next we investigate the reverse process. We start with a skyrmion in the wide part of the nanowire (that is, the right half of the nanowire): see Fig. 1d . We apply a spin-polarized current from left to right. The skyrmion moves from right to left and is converted to a DW pair as it cannot exist in the narrow nanowire whose width is less than 2 R . This result shows that a conversion between a skyrmion and a DW pair is a reversible process ( Supplementary Movie 2 ). We proceed to study the case where we start with a DW pair in the left part of the nanowire whose width is larger than 2 R in Fig. 1g . A skyrmion is created in a similar way as in Fig. 1a , except that the created skyrmion in the junction is greatly deformed. It takes much more time than the previous case ( Fig. 1a ) before the skyrmion changes its shape to its intrinsic size ( Supplementary Movie 3 ). An interesting situation occurs when we consider the reverse process ( Fig. 1j and Supplementary Movie 4 ). A skyrmion is not converted into a DW pair but remains to be a skyrmion when it enters the left part of the nanowire from the right part. The conversion does not occur as the width of the left part of the nanowire is larger than 2 R . Let us describe the conversion process from a DW pair to a skyrmion in detail. First, we start with a DW pair in the narrow part of the nanowire: see Fig. 2a . As the electrical current is applied from the right to the left, the DW pair moves in opposite direction of the applied current. When the right DW reaches the interface, both the end points of the DW are pinned at the junction interface, whereas the central region of DW continues to move. As a result, the DW is deformed into a curved shape: see Fig. 2b . Next, the anti-DW also reaches the junction, and a skyrmion-like structure is formed. This structure still touches the edge at t =0.42 ns ( Fig. 2d ), and then it is decoupled from the edge at t =0.44 ns ( Fig. 2e ). The topological number is not exactly one because of the interference between the skyrmion halo and the edge ( Fig. 2e ). Finally, the skyrmion size shrinks to the intrinsic radius, and the resultant structure becomes a perfect circular shape with Q =1 ( Fig. 2f ). 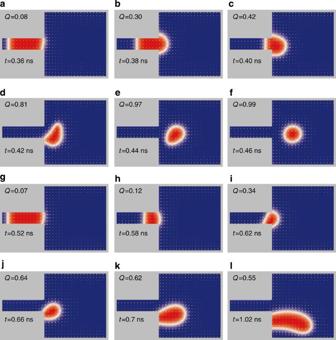Figure 2: Spin configurations of a skyrmion, a meron and a DW pair. (a–f) A skyrmion is created from a DW pair driven by spin transfer torque from the narrow part to the wide part of the nanowire. The spin direction is shown by yellow arrow. A yellow dot in the blue region shows that the spin is almost up, whereas a yellow dot in the red region shows that it is almost down. No dots are observed when the spin is almost perfectly up or down. The in-plane current density along −xdirection is 1.8 μA nm−2in the wide part. (g–l) A meron is created when the in-plane current density along −xdirection is 0.9 μA nm−2in the wide part. Figure 2: Spin configurations of a skyrmion, a meron and a DW pair. ( a – f ) A skyrmion is created from a DW pair driven by spin transfer torque from the narrow part to the wide part of the nanowire. The spin direction is shown by yellow arrow. A yellow dot in the blue region shows that the spin is almost up, whereas a yellow dot in the red region shows that it is almost down. No dots are observed when the spin is almost perfectly up or down. The in-plane current density along − x direction is 1.8 μA nm −2 in the wide part. ( g – l ) A meron is created when the in-plane current density along − x direction is 0.9 μA nm −2 in the wide part. Full size image Meron generation If the applied current density is reduced, the result is dramatically changed as shown in Fig. 2g–l . For smaller current density, a skyrmion is not formed. The critical current density for skyrmion generation is about 1.8 μA nm −2 in the wide part, below which the spin texture is attached to one edge of the nanowire and is elongated ( Fig. 2l ). In this case, the applied current density is 0.9 μA nm −2 in the wide part. The topological number is almost one half, implying that the structure is a meron [20] , which is a half-skyrmion. String geometry It is intriguing to recapitulate the conversion mechanism between a DW pair and a skyrmion in terms of a string geometry. The bulk is separated into two regions with m z >0 (blue) and m z <0 (red) by the boundary with m z =0 (white): see Fig. 2 . The spin direction is almost perpendicular at the skyrmion boundary (defined as m z =0) because of the DMI effect. The boundary may be referred to as a string. A string is either closed or open. It has no branches. An open string must touch the edge. A DW pair consists of two parallel open strings, where the spin directions imply that Q =0. We may argue that there are only two possibilities how these two open strings develop. In the first case, one open string reaches the edge and is expelled ( Fig. 2b ). Then it makes a semicircle. When the other open string reaches the interface separating the narrow part and the wide part of the nanowire, two open strings can form one closed string. The spin direction of a closed string must form a hedgehog with Q =1. It develops into a skyrmion. In the second case, when the velocity is small, an open string may cant near the interface ( Fig. 2h ). The upper part of the DW breaks away from the narrow part of the nanowire, whereas the bulk of the spins is attached to the lower end point ( Fig. 2i) , leading to an open string in the end ( Fig. 2j ). It develops into a meron. Non-topological magnetic solitons without DMI The DMI has two roles. First, the Hamiltonian without the DMI is invariant under the reflection y ↦ − y . Hence, the asymmetric behavior of a skyrmion in Fig. 2 is due to the DMI. The spin configuration forming a hedgehog is also due to the DMI. Second, a skyrmion is stabilized dynamically by the DMI [16] , [17] . Although the topological number Q is defined even without the DMI, it does not have any role if a hedgehog spin configuration is not formed to generate Q =1. To clarify the important roles of the DMI, we have simulated the above process without the DMI. 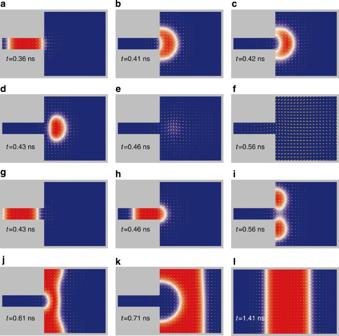Figure 3: Magnetic droplet soliton without DMI. A similar process to Fig. 2 but without the DMI. (a–f) A magnetic droplet soliton is formed from a DW pair, and then disappears by emitting spin waves. It has zero topological number (Q=0). The in-plane current density along −xdirection is 1.8 μA nm−2in the wide part. (g–l) A DW pair remains as a DW pair when the in-plane current density along −xdirection is 1.2 μA nm−2in the wide part. Figure 3a–f shows a similar process to Fig. 2a–f in the absence of the DMI. The magnetization configuration has zero Pontryagin number, implying that the resultant structure is a non-topological magnetic droplet soliton [41] , [42] . The spins of the droplet precess in phase (except for local perturbations) and therefore has a zero Pontryagin number, which can be dynamically stabilized by STT and damping [41] , [42] . Because of the dissipation, the magnetic droplet soliton decays after it breaks away from the interface as it is neither stabilized dynamically nor topologically in this case. Spin waves are emitted when the droplet is damped out, as is shown in Fig. 3f . Figure 3: Magnetic droplet soliton without DMI. A similar process to Fig. 2 but without the DMI. ( a – f ) A magnetic droplet soliton is formed from a DW pair, and then disappears by emitting spin waves. It has zero topological number ( Q =0). The in-plane current density along − x direction is 1.8 μA nm −2 in the wide part. ( g – l ) A DW pair remains as a DW pair when the in-plane current density along − x direction is 1.2 μA nm −2 in the wide part. Full size image Figure 3g–l shows a similar process to Fig. 2g–l in the absence of the DMI when the current density is small. In this case, a DW pair remains as a DW pair but with larger width after some perturbative modulations (see Fig. 3l ). Skyrmion racetrack In the above, the initial state of the simulations all start with a given spin configuration that is, either a DW pair or a skyrmion. For practical applications, it is desirable to create a skyrmion from a ferromagnetic ground state. We apply a periodic modulation of magnetic field, B ( t )= B 0 sin ωt , close to the left edge of the nanowire. The AC field amplitude is B 0 =1 T with frequency of ω =2.5 GHz. A sequence of DWs are created at a regular interval and then deformed into skyrmions. The micromagnetics simulation results are shown in Fig. 4 ( Supplementary Movie 5 ). The total Pontryagin number takes large value corresponding to the creation of skyrmions. This concept can be extended to a skyrmion array if we make multiple nanowires in parallel and then merge into an extended thin film with larger width as shown in Fig. 4b ( Supplementary Movie 6 ). 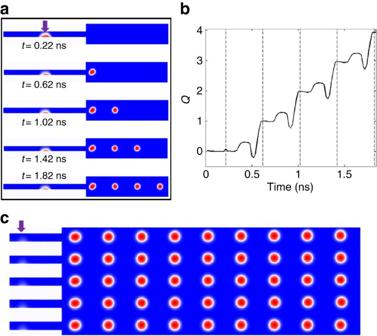Figure 4: Skyrmion racetrack. (a) Top-view of the spin structure at five different times of the simulation, corresponding to the five vertical lines inb. (b) Time-evolution of the topological numberQ. (c) Skyrmion array generations.Qincreases by one unit as one skyrmion is created. The purple arrow represents the position where an external radio-frequency magnetic field is applied to generate DW pairs at a constant time interval. Figure 4: Skyrmion racetrack. ( a ) Top-view of the spin structure at five different times of the simulation, corresponding to the five vertical lines in b . ( b ) Time-evolution of the topological number Q . ( c ) Skyrmion array generations. Q increases by one unit as one skyrmion is created. The purple arrow represents the position where an external radio-frequency magnetic field is applied to generate DW pairs at a constant time interval. Full size image We have presented a conversion mechanism between a DW pair and a skyrmion ( Fig. 2a–f ). We have shown that there exists a critical current density below which a DW pair is converted into a meron ( Fig. 2g–l ) rather than a skyrmion. Without the DMI, the non-topological droplet-soliton ( Fig. 3a–f ) will be generated in the same system. These intriguing results suggest that the proposed nanowire system may provide an excellent environment for studying a wide range of exotic nano-magnetic phenomena, such as skyrmions, DWs and non-topological droplets and so on. The continuous deformation between topologically inequivalent skyrmions and DWs may not only add an additional degree of freedom but also introduce new functionalities for ultradense memory and spin logic applications. A hybrid device ( Fig. 5 ) comprised of skyrmions and DW pairs will have the combined functionalities of individual DW and skyrmion. As illustrated in Fig. 5 , a train of DWs can be generated by applying a field or a current pulse. The information (that is, a series of bit) can be encoded as a train of DWs, which will propagate along the nanowire driven by an external magnetic field or in-plane current, and then will be converted into a train of skyrmions in the channel. In this skyrmion channel, a functional manipulation of skyrmions is to be implemented, which is beyond the scope of the present work. In the drain, skyrmions can be converted back to DWs, enabling read-out of the information encoded in the carrier through the giant-magnetoresistance or tunnelling magnetoresistance effects. A precise control of the time sequence of multi-skyrmions (or skyrmion array) is possible by controlling the magnetic field to create a sequence of DW pairs. Therefore, such hybrid device has the advantages in a number of ways—writability, transmission, power consumption, reliability and readout of the information. 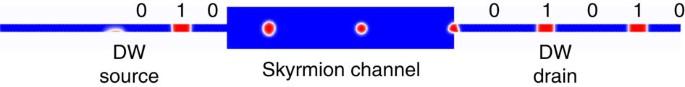Figure 5: A hybrid device based on DWs and skyrmions. A sequence of information (that is, data bits) is encoded as a train of DWs and then converted into a train of skyrmions, which are transmitted in the skyrmion channel. We read out the information by converting the skyrmions back to DWs. The length of the nanowire is 1,600 nm, which is divided into three equal parts, that is, the DW source, the skyrmion channel and the DW drain. Figure 5: A hybrid device based on DWs and skyrmions. A sequence of information (that is, data bits) is encoded as a train of DWs and then converted into a train of skyrmions, which are transmitted in the skyrmion channel. We read out the information by converting the skyrmions back to DWs. The length of the nanowire is 1,600 nm, which is divided into three equal parts, that is, the DW source, the skyrmion channel and the DW drain. Full size image The nucleation of isolated skyrmions is a challenging task as it necessarily involves overcoming the topological barrier [2] , [3] , [21] . In contrast, a variety of writing schemes have been demonstrated to generate a desired pattern of DWs by applying magnetic field only or current pulse through STT effect [26] , [27] , [43] . Therefore, a variety of techniques for DW injection into nanowire has been well-studied [26] , [27] , [43] , [44] , [45] . In this regard, it is more efficient to encode the information in the DW sequence in the source ( Fig. 5 ) as a DW-based device has relatively better writability performance than skyrmions. The maximum velocity of DWs (a few hundred m s −1 up to a few km s −1 ) [46] is approximately at the same order as that of skyrmions (for example, in Fig. 1a , the skyrmion velocity is about 220 m s −1 for an in-plane current density of 1.8 μA nm −2 in the wide part), provided the applied current density exceeding the threshold values for both cases. However, it is shown that the pinning effect for skyrmions motion is much weaker, leading to better mobility and controllability of skyrmions than DWs [3] , [47] . Therefore, it is more efficient to develop an information transmission channel based on skyrmions. In addition, the spacing between skyrmions can be just a few tens of nanometers, which is much smaller than the DWs in racetrack memory [2] , enabling ultradense information storage and transmission based on such hybrid device. One challenging task of spintronics community is to reduce the power consumption and improve the energy efficiency. The critical current density for driving the skyrmions (10 −7 −10 −6 μA nm −2 ) is 4–5 orders smaller than the critical current density for moving DWs (10 −3 −1 μA nm −2 ) [11] , [47] . As shown in Supplementary Figs. 10,11 and 16 , the current density can be greatly reduced for rounded edge geometry, rough interfaces and for sharp turning angle of the interface connecting the two nanowires. In addition, it is possible to further reduce the power consumption by using a much smaller current density to move the skyrmions after the DW pair is converted into skyrmion, which is shown in the Supplementary Note 6 and Supplementary Figs 14–16 . The stability of skyrmions is protected topologically once they are created [3] . Therefore, it is superior to transmit information in the channels based on skyrmions as shown in Fig. 5 . The readout of both skyrmions and DWs can be realized by the giant-magnetoresistance or tunnelling magnetoresistance effect. However, only a small fraction of spins in the skyrmion core are reversed for generating magnetoresistance signal. Therefore, the readout of DW may be advantageous as it makes use of all the fully reversed spins inside the DW. Micromagnetics simulations In the micromagnetics simulations, we have additionally included the DDIs in all numerical calculations [39] . However, the results remain quantitatively the same as those without the DDI. The magnetostatic field at site i can be described as where r ik = r k − r i . We have numerically solved the Landau–Lifshitz–Gilbert equation by fourth-order Runge–Kutta method at T =0 K. For finite temperature simulations ( T =300 K) shown in the Supplementary Fig. 13 , we use the Heun scheme and a fixed time step of 0.1 fs in the simulation. All simulations have been checked by the open source micromagnetics simulation codes OOMMF and Mumax, which give very similar results [48] , [49] . Derrick–Hobart theorem The dynamical stability of a skyrmion is given by the Derrick–Hobart theorem [50] , [51] by examining the scaling property. The Hamiltonian consists of the the nonlinear O(3) sigma model H X describing the exchange energy, the easy-axis anisotropy term H A , the DMI term H DM and the Zeeman term H Z . Suppose there exists a soliton solution n 0 ( x ) to the system, we calculate each contribution as , , and . Now we consider the configuration n ( x )= n 0 ( λx ). Substituting this into each term, we find the energy of the new configuration to be This function has a unique minimum point at where λ =1 for consistency. The scale is uniquely fixed. From this theorem, it is clear that a soliton solution is stabilized by the DMI. On the other hand, we find that λ →∞ as from equation (5), which implies that a soliton shrinks to zero without the DMI. How to cite this article: Zhou, Y. and Ezawa, M. A reversible conversion between a skyrmion and a domain-wall pair in a junction geometry. Nat. Commun. 5:4652 doi: 10.1038/ncomms5652 (2014).